Highly efficient methane biocatalysis revealed in a methanotrophic bacterium Methane is an essential component of the global carbon cycle and one of the most powerful greenhouse gases, yet it is also a promising alternative source of carbon for the biological production of value-added chemicals. Aerobic methane-consuming bacteria (methanotrophs) represent a potential biological platform for methane-based biocatalysis. Here we use a multi-pronged systems-level approach to reassess the metabolic functions for methane utilization in a promising bacterial biocatalyst. We demonstrate that methane assimilation is coupled with a highly efficient pyrophosphate-mediated glycolytic pathway, which under oxygen limitation participates in a novel form of fermentation-based methanotrophy. This surprising discovery suggests a novel mode of methane utilization in oxygen-limited environments, and opens new opportunities for a modular approach towards producing a variety of excreted chemical products using methane as a feedstock. Nature provides two alternative forms of methane as a resource: natural gas, relatively abundant today but still a non-renewable fossil fuel, and renewable biogas, a byproduct of modern society that is often wasted [1] , [2] , [3] . Interest in new technologies for effective conversion of flared/waste sources of methane into chemical compounds, including next-generation fuels, continues to increase [4] , [5] , [6] . The use of microbial cells and enzymes as catalysts for methane conversion represents an appealing approach in this context [7] , [8] , [9] , [10] , [11] . The benefits of methane biotechnology include a self-sustainable component, as any biomass generated could be used as single cell protein or converted back to methane via anaerobic digestion. However, besides single cell protein and polyhydroxybutyrate, exploitation of methane-based catalysis for the production of chemicals and fuels has not yet proven successful at the commercial level. Gammaproteobacterial methanotrophs with the ribulose monophosphate (RuMP) pathway are among the most promising microbial systems for methane-based biotechnology. Reconstruction of the methane utilization network in these methanotrophs has been based on a number of biochemical studies that pointed towards the Entner–Doudoroff (EDD)-variant of the RuMP pathway as the major route for single carbon (C 1 ) assimilation [12] , [13] , [14] . The major biochemical evidence that favoured the EDD variant of the RuMP cycle included relatively high activities of two key enzymes of the pathway (6-phosphogluconate dehydratase and 2-keto-3-deoxy-6-phosphogluconate aldolase) and multiple enzymatic lesions in the Embden–Meyerhof–Parnas (EMP) pathway [15] , [16] . Activity of pyruvate kinase has not been detected previously in any gammaproteobacterial methanotroph [16] , [17] . The presence of a reversible pyrophosphate (PPi)-dependent phosphofructotransferase led to the conclusion that the EMP pathway represents a metabolic loop balancing the level of glyceraldehyde-3-phosphate and phosphoenolpyruvate (PEP) [16] , [18] . This metabolic arrangement has served as the foundation for theoretical characterization of efficiency and yield of methane utilization [14] , [15] . However, the predicted maximum carbon conversion efficiency (39–47%) was considerably less than measured values (64–66.5%) [15] , [19] . Theoretically, the RuMP pathway can provide a better efficiency of carbon utilization when operated via the EMP pathway than via the EDD pathway [14] . Genomic studies indicate that a complete set of EMP pathway enzymes is encoded in the genomes of all sequenced methanotrophic bacteria harbouring the RuMP pathway for methane assimilation. Furthermore, proteomic studies showed that both pathways are expressed in Methylococcus capsulatus [20] . In this work, we renew the current understanding of metabolic functions essential for methane utilization through detailed investigations of C 1 -assimilation in Methylomicrobium alcaliphilum strain 20Z, a haloalkalitolerant methanotroph that is a promising biocatalyst [11] . Availability of the M. alcaliphilum 20Z genome sequence [21] allowed us to apply systems-level approaches including genome-wide transcriptomic studies (Illumina-based RNA-Seq), metabolomics and 13 C-label distribution analysis of methane-grown cultures for metabolic reconstruction of C 1 utilization pathways in this strain. Transcriptomic study M. alcaliphilum 20Z grown aerobically with methane as the sole source of carbon and energy showed high levels of expression for genes known to be involved in the metabolism of C 1 compounds including those for membrane-bound methane monooxygenase ( pmoCAB ), PQQ-dependent methanol dehydrogenase ( mxaFIG ) and two key enzymes of the RuMP pathway-hexulose phosphate synthase ( hps ) and phosphohexuloisomerase ( hpi ) ( Fig. 1a ; Supplementary Table S1 ), as expected. The relative abundance of transcripts for enzymes involved in the RuMP pathway downstream from fructose-6-phosphate were 3–20-fold lower than those of hpi and hps . Remarkably the abundance of transcripts encoding glycolytic pathway enzymes was 2–10-fold higher than EDD pathway enzymes (that is, edd and eda ) ( Supplementary Table S1 ). Furthermore, one of the putative pyruvate kinase genes, pyk2 (MALCv4_3080), showed high expression. 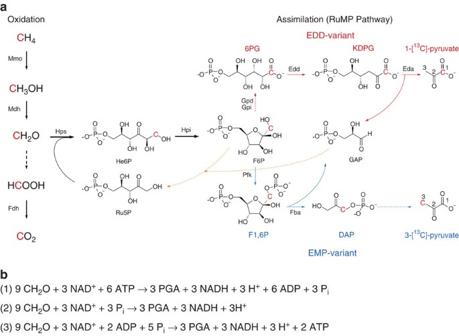Figure 1: Methane oxidation and formaldehyde assimilation. (a) Predicted positions of incorporated13C (indicted in red) for the EDD (dark red arrows) and the EMP (blue arrows) variants. Dashed lines indicate multistep reactions. The pentose-phosphate pathway variant for regeneration of ribulose 5-phosphate is indicated by orange dashed arrows. Enzyme activities (in nmol min1per mg protein) in cell free extracts ofM. alcaliphilum20Z were as follows: methane monoxygenase (Mmo), 70±5; PQQ-dependent methanol dehydrogenase (Mdh), 230±12; NAD-dependent formate dehydrogenase (Fdh), 130±7; hexulose phosphate synthase/hexulose phosphate isomerase (Hps/Hpi), 600±30; glucose phosphate isomerase (Gpi), 32±5; NADP-dependent glucose 6-phosphate dehydrogenase, 34±2 (Gpd); NAD-dependent glucose 6-phosphate dehydrogenase, 23±2 (Gdp); NADP-dependent 6-phosphogluconate dehydrogenase (Edd), 32±2; KDPG aldolase (Eda), 60±4; fructose-bisphosphate aldolase (Fba), 35± 2; PPi-phosphofructokinase (Pfk), 70± 4. (b) Summary equations for production of 3-phosphoglycerate from formaldehyde via the RuMP pathway for the EDD variant (1) or the EMP variant with either the ATP-dependent EMP pathway (2) or the PPi-dependent EMP pathway (3). Abbreviations: Ru5P, ribulose 5-phosphate; He6P, 3-hexulose 6-phosphate; F6P, fructose 6-phosphate; KDPG, 2-keto-3-deoxy 6-phosphogluconate; F1,6P, fructose 1,6-bisphosphate; DAP, dihydroxyacetone phosphate; GAP, glyceraldehyde 3-phosphate; PGA, 3-phosphoglycerate; Pi, inorganic phosphate. Figure 1: Methane oxidation and formaldehyde assimilation. ( a ) Predicted positions of incorporated 13 C (indicted in red) for the EDD (dark red arrows) and the EMP (blue arrows) variants. Dashed lines indicate multistep reactions. The pentose-phosphate pathway variant for regeneration of ribulose 5-phosphate is indicated by orange dashed arrows. Enzyme activities (in nmol min 1 per mg protein) in cell free extracts of M. alcaliphilum 20Z were as follows: methane monoxygenase (Mmo), 70±5; PQQ-dependent methanol dehydrogenase (Mdh), 230±12; NAD-dependent formate dehydrogenase (Fdh), 130±7; hexulose phosphate synthase/hexulose phosphate isomerase (Hps/Hpi), 600±30; glucose phosphate isomerase (Gpi), 32±5; NADP-dependent glucose 6-phosphate dehydrogenase, 34±2 (Gpd); NAD-dependent glucose 6-phosphate dehydrogenase, 23±2 (Gdp); NADP-dependent 6-phosphogluconate dehydrogenase (Edd), 32±2; KDPG aldolase (Eda), 60±4; fructose-bisphosphate aldolase (Fba), 35± 2; PPi-phosphofructokinase (Pfk), 70± 4. ( b ) Summary equations for production of 3-phosphoglycerate from formaldehyde via the RuMP pathway for the EDD variant (1) or the EMP variant with either the ATP-dependent EMP pathway (2) or the PPi-dependent EMP pathway (3). Abbreviations: Ru5P, ribulose 5-phosphate; He6P, 3-hexulose 6-phosphate; F6P, fructose 6-phosphate; KDPG, 2-keto-3-deoxy 6-phosphogluconate; F1,6P, fructose 1,6-bisphosphate; DAP, dihydroxyacetone phosphate; GAP, glyceraldehyde 3-phosphate; PGA, 3-phosphoglycerate; Pi, inorganic phosphate. Full size image Characterization of methanotrophic pyruvate kinase In accordance with previous studies, no pyruvate-forming activity was detected in cell-free extracts of M. alcaliphilum strain 20Z with three different enzymatic assays (see Methods). However, when the pyruvate kinase gene was overexpressed in Escherichia coli , purified protein preparations displayed significant pyruvate kinase activity (7 U mg −1 of protein at the optimum pH 7.5) ( Table 1 and Supplementary Table S2 ). We found that the enzyme activity was strongly stimulated (20-fold) in the presence of a set of the RuMP pathway intermediates: glucose-6-phosphate, fructose-6-phosphate, ribose-5-phosphate, ribulose-5-phosphate or erythrose-4-phosphate ( Supplementary Table S2 ). ATP, PPi and Pi strongly inhibited enzyme activity; however, this inhibitory effect was completely abolished by the addition of activators such as fructose-6-phosphate or ribose-5-phosphate. Overall, the data suggest that the strain possesses an active pyruvate kinase that is strongly dependent on the presence of RuMP cycle intermediates. It should be mentioned that the pyruvate kinase does not show any activity in cell extracts from methanotrophic bacteria, even after supplementation with the inducers shown in Table 1 and Supplementary Table S2 . As pyk2 is one of the highly expressed genes in the transcriptome of strain 20Z, and the protein is readily detected (Kalyuzhnaya, unpublished data), we can only speculate that in methanotrophs the enzyme is not stable or is inactivated by another yet unknown component, such as a tightly bound inhibitor, a protease or a modifying protein. However, the kinetic properties of Pyk2 indicate that significant flux of cell carbon could occur via the EMP pathway in methanotrophic bacteria. In order to further test this hypothesis, we analysed the intracellular concentrations of pathway intermediates using a metabolomic approach. Table 1 Kinetic characteristics of pyruvate kinase 2 from M. alcaliphilum 20Z. Full size table EMP pathway is the main route for C 1 -carbon assimilation In cells of M. alcaliphilum 20Z grown on methane, the intracellular abundance of the majority of EMP pathway intermediates is high ( Supplementary Table S3 ). In contrast, two key intermediates of the EDD pathway, 6-phosphogluconate and 2-dehydro-3-deoxy-phosphogluconate were only barely detected in cell samples. To further probe the metabolic pathway for methane assimilation in M. alcaliphilum 20Z, we monitored the dynamic incorporation of 13 C-labelled methane into downstream intermediates of the RuMP pathway ( Supplementary Fig. S1 ). As expected, the relative abundance of fructose 6-phosphate/glucose 6-phosphate increased at very early time points, demonstrating that methane was rapidly assimilated through the reaction of Ru5P and 13 C-labelled formaldehyde. The downstream metabolites phosphoglycerate and PEP were also sequentially labelled. Owing to the low pool size, we were not able to estimate the rate of incorporation of 13 C-carbon into intermediates of the EDD pathway. In order to distinguish between the two pathways, we performed 13 C-pyruvate tracing analysis coupled with tandem mass spectrometry. If pyruvate is formed via the EDD pathway, the initial 13 C-incorporation should be observed in position 1; in contrast, pyruvate derived from PEP through the EMP pathway should be labelled in position 3 ( Fig. 1a ). As shown in Fig. 2 , only a small fraction of pyruvate was labelled in position 1 during the course of the experiment. The rate of 13 C incorporation into position 3 of pyruvate was at least six-fold higher than the rate of incorporation into position 1. These experiments confirmed that the major fraction of cellular pyruvate comes from the EMP pathway during growth of the methanotrophic culture on methane. A similar carbon isotopic distribution in pyruvate was observed for Methylomonas sp. LW13, a typical representative of gammaproteobacterial methanotrophic bacteria ( Supplementary Fig. S2 ). 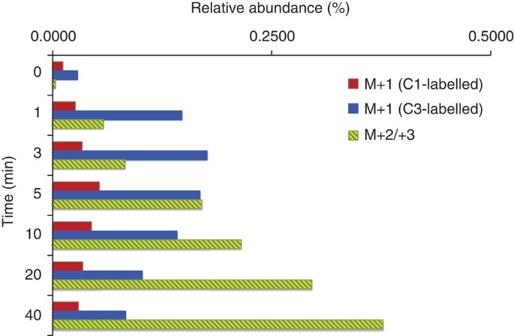Figure 2: Pyruvate13C-labelling patterns inM. alcaliphilum20Z. Intracellular pyruvate was resolved by multiple reactions monitoring scan mode on mass spectrometry. Green,13C-doubly and triply labelled pyruvate; red,13C-pyruvate labelled in position 11; Blue,13C- pyruvate labelled in position 33. Figure 2: Pyruvate 13 C-labelling patterns in M. alcaliphilum 20Z. Intracellular pyruvate was resolved by multiple reactions monitoring scan mode on mass spectrometry. Green, 13 C-doubly and triply labelled pyruvate; red, 13 C-pyruvate labelled in position 1 [1] ; Blue, 13 C- pyruvate labelled in position 3 [3] . Full size image Methane utilization via fermentation The new arrangement of the methanotrophic network opens up a possibility for fermentation. Methanotrophs require O 2 for the oxidation of methane, so experiments were carried out with cells grown in bioreactors in which air was provided at low levels and the dissolved O 2 concentrations were kept at undetectable to 0.1%. In a continuous bioreactor culture, M. alcaliphilum 20Z grew slowly, with a doubling time of 23 h. Transcriptomic profiles of batch bioreactor cultures grown at low O 2 showed that similar to what is observed for aerobic growth, relative expression of EMP genes is high. The most notable changes in the transcriptome were the downregulation of genes for NADH:ubiquinone oxidoreductase and cytochrome c oxidase, and the upregulation of genes for the O 2 carrier bacteriohemerythrin and for the pathways for mixed-acid fermentation and H 2 production ( Supplementary Table S1 and Supplementary Fig. S3 ). In our experiments, the expression profile of bacteriohemerythrin, shown to be essential for high in vitro activity of particulate methane monooxygenase in M. capsulatus Bath [22] , indicated that it most likely contributes to O 2 -scavenging/partitioning in M. alcaliphilum 20Z. Genes predicted to encode fermentation pathway enzymes with increased expression under microoxic conditions included a putative acetate kinase, 3-ketoacyl-CoA thiolase, 3-hydroxyacyl-CoA dehydrogenase, malate dehydrogenase, fumarase, succinate dehydrogenase and lactate dehydrogenase. Intriguingly, upregulation of genes encoding a NAD-reducing hydrogenase was observed ( Supplementary Table S1 ). These changes suggested production of a set of possible fermentation products, including formate, acetate, succinate, lactate, 3-hydroxybutyrate and H 2 . Significantly, in bioreactor cultures acetate, succinate, lactate and H 2 were detected, but only in medium from batch and chemostat cultures grown at low O 2 tension, whereas formate increased about threefold ( Table 2 ). Extracellular concentrations of these acids increased markedly after incubation of low O 2 bioreactor samples in closed vials flushed with N 2 . Low amounts of 3-hydroxybutyrate also accumulated. Furthermore, significant accumulation of H 2 was detected in closed vial experiments ( Table 2 ). Similar incubations supplied with 13 C-methane confirmed that formic and acetic acids were produced from methane ( Supplementary Table S4 ). The rate of methane consumption in the closed vial experiments was exceptionally low (1.75±0.41 nmol min −1 per mg protein −1 ); however 3% and 15% of the added methane was consumed in 12 and 60 h, respectively. The total amount of produced extracellular carbon, mostly acetate and formate, was equivalent to 40–50% of the total methane carbon consumed. These data suggest that in the presence of sufficient O 2 to drive methane oxidation, M. alcaliphilum 20Z is capable of fermentation from methane-derived formaldehyde, and that methane utilization at low O 2 tension involves switching to a novel fermentation mode leading to the formation of formate, acetate, succinate, lactate and hydroxybutyrate as end products, with little biomass synthesis ( Fig. 3 ). The presence of putative fermentation genes in the genome of gammaproteobacterial methanotrophs suggests that this type of metabolism is likely widespread ( Supplementary Table S5 ). Table 2 Accumulation of extracellular metabolites ( μ mol (g DCW −1 )). 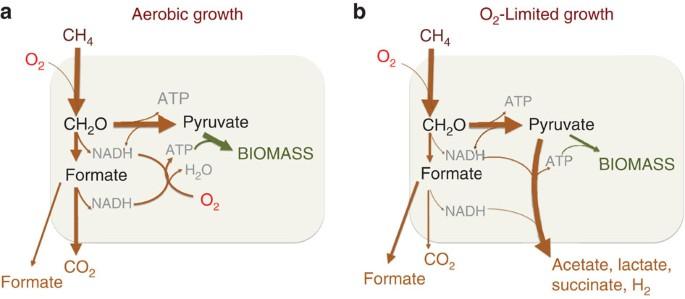Figure 3: Proposed schemes for methane utilization inM. alcaliphilum20Z. (a) Methane utilization at O2saturation; (b) Methane utilization at O2-limiting conditions. Full size table Figure 3: Proposed schemes for methane utilization in M. alcaliphilum 20Z. ( a ) Methane utilization at O 2 saturation; ( b ) Methane utilization at O 2 -limiting conditions. Full size image The experiments presented here change our understanding of methane assimilation through the RuMP pathway in obligate methanotrophic bacteria in some fundamental aspects. First, utilization of the PPi-mediated EMP pathway significantly increases the predicted efficiency of one-carbon assimilation. Genes encoding a membrane-bound proton-translocating pyrophosphatase show significant expression, suggesting that this enzyme could be one of the possible candidates for the regeneration of PPi from ATP. The predicted ratio of ATP hydrolysis/PPi formation for this class of enzymes is 1:3 (ref. 23 ). Therefore, not only does the assimilation of 9 mol of formaldehyde by this metabolic scheme to generate three 3-carbon intermediates require no additional energy, it actually produces three moles of reducing power (NADH) and two moles of ATP ( Fig. 1b ). Second, the surprising discovery of this ATP-producing assimilatory route raised the possibility of fermentation as a new mode of methane utilization. The ability of methanotrophic cultures to convert methane into excreted organic compounds has previously been described and it has been suggested to support denitrification by wastewater treatment communities [19] , [24] , [25] , [26] , [27] . However, metabolic pathways for production of organic compounds from methane were unknown, and excreted compounds were often described as the product of cell lysis or a starvation response [24] , [25] , [26] , [27] . Our results suggested the possibility that organic acids could be produced as a result of fermentation. This discovery challenges our understanding of methanotrophy as microbial metabolism linked to respiration (O 2 , NO 3 − or SO 4 2− ) and has major implications for the environmental role of methanotrophic bacteria in removing this greenhouse gas in O 2 -limited environments. Numerous environmental studies indicate that gammaproteobacterial methanotrophs thrive at oxic–anoxic interfaces [28] , [29] , [30] . If fermentation is the major metabolic mode of methane cycling under O 2 -limiting conditions, then our understanding of the role of methanotrophic bacteria in supporting the global carbon cycle may be in need of revision in some respects – not so much in terms of carbon being mineralized into CO 2 , but of the proportion of carbon ending in biomass ( Fig. 3 ). Most notably, in our experiments, only a small fraction of the oxidized methane was converted to biomass, so methanotrophic bacteria may represent only a minor part of the overall microbial community involved in the conversion of methane into biomass. Rather, our results suggest the possibility that in O 2 -limiting environments, methanotrophs drive the conversion of methane to excreted products and hydrogen, which are then used and transformed by non-methanotrophs. If confirmed by future work, this has implications for microbial community structure and functioning in environments where the methane cycle is prominent. The surprising discovery of glycolysis-based methane assimilation and production of hydrogen in strain M. alcaliphilum 20Z may open new opportunities to producing a variety of products using methane as a feedstock, provided this pathway may be operated in a sufficiently efficient way in the laboratory. Virtually all biosynthetic modules for the production of a wide variety of chemicals developed for glucose-based catalysis in E. coli could also be implemented in cultures containing this EMP variant of the RuMP pathway. Thus, our demonstration of methane-based fermentation suggests new approaches for the commercial conversion of methane to hydrogen and excreted products using microoxic production conditions. Cell cultivation and growth parameters M. alcaliphilum 20Z cells were grown using a mineral salts medium [31] in either closed vials (50 ml culture in 250 ml vials, with shaking at 200 r.p.m.) or bioreactor cultures (fed-batch or chemostat; 1 l working volume in a 2 l bench top BioFlo 110 modular bioreactor, New Brunswick Scientific, Edison, NJ, USA). Cells were grown at 28 o C. Optical density of cell cultures was measured on a Beckman DU 640B spectrophotometer in plastic 1.5 ml cuvettes with a 1 cm path length. Chemostat cultures maintained a steady-state optical density at 600 nm (OD 600 ) of ~2.0±0.2. The dilution rate was 0.12 h −1 for aerobic cultures (influent gas mixture – 20% CH 4 :20% O 2 :60 N 2 , dissolved O 2 tension was 49–54%) and 0.03 h −1 for low O 2 cultures (influent gas mixture 20% CH 4 :5% O 2 :75 %N 2 ; dissolved O 2 tension was non-detectable to 0.1%. pH (9.0) was controlled by the automatic addition of 1N NaOH. Agitation was kept constant at 1000 r.p.m. Samples of inflow and outflow gases were collected daily in triplicates for gas analysis. The rates of methane consumption and H 2 production were determined by incubating cell samples (50 ml, OD 600 between 2 and 4) in closed 250 ml vials for 12–60 h at 28 °C. Before incubation, vials were flushed for 15 min with a gas mixture containing either 20% CH 4 :5% O 2 :75% N 2 or 20% CH 4 :80% N 2 , or 20% 13 CH 4 :80%N 2 . Gas analysis Methane measurements were made on a Shimadzu Gas Chromatograph GC-14A, using an FID detector with helium as the carrier gas. O 2 and H 2 measurements were made on a multiple gas analyser SRI 8610C Gas Chromatograph equipped with TCD/FID detectors (SRI Instruments). Concentrations of gases were deduced from standard curves. Gene expression RNA extraction, sequencing, alignment and mapping were performed as described [32] . Metabolite measurement Metabolic and 13 C-labelling studies on batch and fed-batch cultures were carried out as described [33] with modification for desalting. Briefly, the dried sample was re-dissolved in 1 ml water and handled according to SPE procedures [34] . MCX, MAX and WAX cartridges (1 cm 3 , 30 mg, Waters, Milford, MA, USA) were preconditioned separately. A WAX cartridge was connected beneath a MCX cartridge. Each 1 ml sample was directly loaded through both the MCX and WAX reservoirs. The loaded fraction was collected and made basic with 5% ammonium hydroxide and then loaded into a MAX reservoir, followed by elution. After loading and washing with 1 ml of water, the two adjacent MCX and WAX cartridges were disconnected and eluted separately. All the eluted solutions were dried using a vacuum centrifuge. For liquid chromatography-tandem mass spectrometry analysis, each dried sample was re-dissolved in 50 μl water and pooled. Liquid chromatography-tandem mass spectrometry experiments were carried out on a Waters LC-MS system consisting of a 1,525 μ binary HPLC pump with a 2777C autosampler coupled to a Quattro Micro API triple-quadrupole mass spectrometer (Micromass, Manchester, UK), or a Thermo Scientific TSQ quantum access triple-stage quadrupole mass spectrometer. The HILIC columns (Luna NH 2 , 250 mm × 2 mm, 5 μm, and ZIC-HILIC, 150 mm × 4.6 mm, 5 μm) employing gradient elution were carried out using the previously described conditions [35] , [36] . Sugar phosphates were measured by using an ion pairing-reverse phase method [37] . Singly labelled pyruvate position was determined by multiple reaction monitoring (MRM) scan mode with an injection volume of 10 μl. The MRM experiments were carried out as described previously [38] . The dwell time for each MRM transition was 0.08 s. All peaks were integrated using Masslynx Applications Manager (version 4.1) software. Quantification of metabolites was obtained by adding culture-derived global 13 C-labelled internal standards before cell extraction [37] . Relative abundance (%) was obtained by normalizing the pool of each metabolite to the sum of all the targeted metabolites. Dynamic 13 C incorporation For the 13 C methane tracing experiment, M. alcaliphilum 20Z cells grown to mid-exponential phase (OD 600 =0.6–0.8) on 12 C methane in vials or fed-batch bioreactor were rapidly transferred to a fresh flask with the same percentage of 13 C methane as the sole carbon source as deduced from a growth curve. At the defined time points, the cell culture was harvested and metabolites were analysed as described above. Protein purification and characterization Activities of key enzymes of central metabolic pathways were measured as described [18] , [39] , [40] . Pyruvate-forming activity in cell-free extracts of M. alcaliphilum 20Z was also measured using Pyruvate Assay Kit (BioVision Inc., CA, USA). Recombinant pyruvate kinase PK-ubiqitin-His 6 was obtained by cloning of the pyk2 gene (MALCv4_3080) in the vector pHUE and expressing in E. coli BL21 (DE3) cells growing in the presence of 0.5 mM IPTG for 5 h at 37 °C. PK-ubiqitin-His 6 enzyme was purified by affinity chromatography on a Ni 2+ -NTA column as described earlier [39] . NMR analysis To estimate the concentration of metabolites excreted into growth medium, 50 ml samples were collected. Cells were separated by centrifugation (15 min at 2,700 × g ), filtration via 0.2 μm filter units followed by ultrafiltration through Amicon@Ultra 3K filters. NMR analyses of the culture media were made using a Bruker AVANCE III 800 MHz or 700 MHz spectrometer equipped with a cryoprobe or a room temperature probe suitable for 1 H inverse detection with Z-gradients at 298 K. The solvent, water, was removed from the 1 ml culture media samples by drying the samples using a rotary evaporator. The residue was dissolved in an equal volume of phosphate buffer prepared in deuterated water (0.1 M; pH = 7.4) containing 0.2 mM TSP (3-(trimethylsilyl) propionic-2,2,3,3-d 4 acid sodium salt). From this solution, 600 μl was placed in a 5 mm NMR tube for analysis. One-dimensional 1 H NMR spectra were obtained using a one pulse sequence that included residual water signal suppression from a pre-saturation pulse during the relaxation delay. For each sample, 32 k data points were acquired using a spectral width of 10,000 Hz and a relaxation delay of 6 s. The data were processed using a spectral size of 32 k points and by multiplying with an exponential window function equivalent to a line broadening of 0.3 Hz. The resulting spectra were phase and baseline corrected and referenced with respect to the internal TSP signal. Metabolite peaks in the spectra were then assigned using chemical shift databases, and the peak areas were obtained by integration. Using these peak areas, along with the known concentration of the internal reference (TSP) and the number of protons each peak represented in the molecule, the metabolite concentrations in the culture media were estimated. Similarly, concentrations for the 13 C labelled bacterial products were estimated using 13 C satellite peaks of metabolites in the 1 H NMR spectra. Bruker Topspin version 3.0 and 3.1 software packages were used for NMR data acquisition and processing, respectively. Accession codes : The RNA-Seq data from this study have been deposited in NCBI’s Gene Expression Omnibus (GEO) database under accession GSE51145 . How to cite this article: Kalyuzhnaya, M.G. et al. Highly efficient methane biocatalysis revealed in a methanotrophic bacterium. Nat. Commun. 4:2785 doi: 10.1038/ncomms3785 (2013).